Absorption-induced scattering and surface plasmon out-coupling from absorber-coated plasmonic metasurfaces Interactions between absorbers and plasmonic metasurfaces can give rise to unique optical properties not present for either of the individual materials and can influence the performance of a host of optical sensing and thin-film optoelectronic applications. Here we identify three distinct mode types of absorber-coated plasmonic metasurfaces: localized and propagating surface plasmons and a previously unidentified optical mode type called absorption-induced scattering. The extinction of the latter mode type can be tuned by controlling the morphology of the absorber coating and the spectral overlap of the absorber with the plasmonic modes. Furthermore, we show that surface plasmons are backscattered when the crystallinity of the absorber is low but are absorbed for more crystalline absorber coatings. This work furthers our understanding of light–matter interactions between absorbers and surface plasmons to enable practical optoelectronic applications of metasurfaces. Plasmonic metasurfaces are emerging as two-dimensional (2D) metamaterials capable of manipulating light on the nanoscale with the possibility of being incorporated into optoelectronic devices. Metasurfaces are typically composed of arrays of sub-wavelength metallic nanostructures where the macroscopic electromagnetic properties of the surface arise from the collective response of the individual nanostructures [1] , [2] , [3] , [4] . This collective response has led to a host of intriguing optical phenomena, such as negative refractive index [5] , [6] and permeability [7] , phase control [8] , [9] , optical cloaking [10] , and electromagnetic field enhancements [11] , [12] . When plasmonic (meta)materials are coated with absorbers, many additional effects have been observed, such as absorption-induced transparency [13] , [14] , strong coupling between plasmons and excitons [15] , [16] , [17] , plasmonic splitting [18] and enhanced absorption within the absorber [15] , [19] , [20] . For practical applications, it is important to understand how the properties of plasmonic metasurfaces are influenced by the presence of semiconductor absorber thin films. Furthermore, besides the unique optical phenomena exhibited by absorber-coated metasurfaces, the effects of morphology and crystallinity of absorber coatings on metasurface optical properties have not been widely considered. Because of their propensity for solution-based deposition and applications for bulk-heterojunction organic photovoltaics (BHJ-OPVs) [21] , [22] , [23] , [24] , [25] and polymer light-emitting diodes (PLEDs) [26] , [27] , [28] , organic semiconductors are practical materials to employ to investigate the interactions between absorbers and plasmonic metasurfaces. Here, we elucidate the optical modes supported by silver plasmonic metasurfaces coated with organic semiconductor absorbers using dark-field (DF) scattered-light spectroscopy. In particular, we identify two interesting optical phenomena that arise from the absorber-coated metasurfaces: a previously unidentified optical mode type called absorption-induced scattering (AIS), and out-coupling of surface plasmon polaritons (SPPs). AIS is shown to originate from electromagnetic coupling between optical transitions of absorber materials and scattering modes, regardless of whether the scattering modes are plasmonic, localized or collective in origin. We then show that the crystallinity of the organic absorber affects out-coupling of SPP modes, with lower crystallinity absorber coatings facilitating greater out-coupling of SPPs. We conclude by showing that these optical modes affect absorption within both the absorber coating and metasurface materials to different extents: localized surface plasmon resonances (LSPRs) contribute more to absorption in the coating than in the metal, while AIS and SPPs are absorbed more by the metasurface. However, total absorption arising from AIS and SPPs is smaller than that for LSPRs. This work serves to highlight a previously unexplored optical scattering phenomenon that occurs from thin-film semiconductor absorber layers and to further our understanding of how to control light–matter interactions at metasurfaces for practical optoelectronic applications. Absorber-coated plasmonic metasurfaces We fabricated large-area disordered plasmonic metasurfaces composed of Ag nanoparticle arrays (AgNPAs) on Ag thin films (that is, AgNPA/Ag) by nanotemplating ( Fig. 1a,c ; Methods). We prepared disordered metasurfaces due to facile large-area fabrication and because random arrays of nanostructures can couple into a larger number of optical modes than periodic arrays [29] , [30] . The collective scattering response of AgNPA/Ag metasurfaces observed by DF imaging was in stark contrast to that of planar Ag films, which exhibited minimal scattering ( Fig. 1b and insets in Fig. 1c,d ). We prepared Ag nanoparticles (AgNPs) with heights of 48.9±9.7 nm, base diameters of 88.3±22.5 nm and an average array period of 145.7±25.8 nm ( Supplementary Fig. 1 ). Organic semiconductor absorber coatings were deposited by spin coating on top of the AgNPA/Ag to a thickness of 72.8±10.4 nm (a thickness that has been used frequently throughout the BHJ-OPV literature [31] , [32] ; Supplementary Figs 2 and 3 ) and partially conformed to the AgNPA/Ag metasurfaces ( Fig. 1e , Supplementary Fig. 4 ). As absorber coatings, we selected three well-known organic conjugated polymers (poly(3-hexylthiophene-2,5-diyl) (P3HT); poly[ N -9’-heptadecanyl-2,7-carbazole- alt -5,5-(4’,7’-di-2-thienyl-2’,1’,3’-benzothiadiazole)] (PCDTBT); poly([4,8-bis[(2-ethylhexyl)oxy] benzo[1,2- b :4,5- b ’]dithiophene-2,6-diyl][3-fluoro-2-[(2-ethylhexyl)carbonyl]thieno[3,4- b ] thiophenediyl]) (PTB7)) and polymer:fullerene active layer systems used for BHJ-OPV devices (P3HT blended with [6,6]-phenyl-C 61 -butyric acid methyl ester (PCBM); PCDTBT blended with [6,6]-phenyl-C 71 -butyric acid methyl ester (PC 70 BM); and PTB7 blended with PC 70 BM). 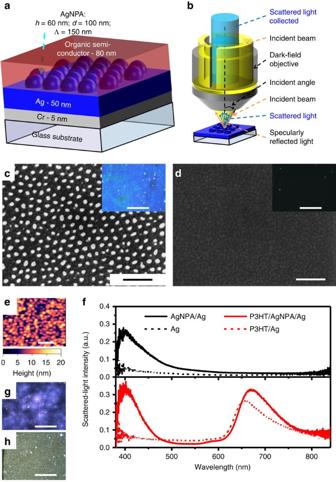Figure 1: Absorber-coated plasmonic metasurfaces. (a) Schematic of a plasmonic metasurface with an organic semiconductor thin-film coating (AgNPA, silver nanoparticle array;h, nanoparticle height;d, nanoparticle diameter; Λ, nanoparticle period). (b) Schematic of the reflection-mode, dark-field (DF) scattered-light imaging and spectroscopy set-up. (c,d) Scanning electron microscope (SEM) images of a Ag film coated with a AgNPA (that is, a plasmonic metasurface) (c) and a planar Ag film (d). Scale bars, 500 nm. Insets are true-colour DF images of the respective films acquired under Xenon lamp illumination; scale bars, 100 μm. (e) Atomic force microscope (AFM) surface topography of a P3HT-coated AgNPA/Ag metasurface. Scale bar, 500 nm. (f) DF scattered-light spectra for AgNPA/Ag metasurfaces and planar Ag films, with and without P3HT coatings. (g,h) True-colour DF images of a P3HT-coated AgNPA/Ag metasurface (g) and a P3HT-coated planar Ag film (h) acquired under Xenon lamp illumination. Scale bars, 100 μm. Figure 1: Absorber-coated plasmonic metasurfaces. ( a ) Schematic of a plasmonic metasurface with an organic semiconductor thin-film coating (AgNPA, silver nanoparticle array; h , nanoparticle height; d , nanoparticle diameter; Λ, nanoparticle period). ( b ) Schematic of the reflection-mode, dark-field (DF) scattered-light imaging and spectroscopy set-up. ( c , d ) Scanning electron microscope (SEM) images of a Ag film coated with a AgNPA (that is, a plasmonic metasurface) ( c ) and a planar Ag film ( d ). Scale bars, 500 nm. Insets are true-colour DF images of the respective films acquired under Xenon lamp illumination; scale bars, 100 μm. ( e ) Atomic force microscope (AFM) surface topography of a P3HT-coated AgNPA/Ag metasurface. Scale bar, 500 nm. ( f ) DF scattered-light spectra for AgNPA/Ag metasurfaces and planar Ag films, with and without P3HT coatings. ( g , h ) True-colour DF images of a P3HT-coated AgNPA/Ag metasurface ( g ) and a P3HT-coated planar Ag film ( h ) acquired under Xenon lamp illumination. Scale bars, 100 μm. Full size image To determine the optical behaviour of the metasurfaces with organic semiconductor absorber coatings, we conducted DF scattered-light spectroscopy in reflection mode using a microscope-coupled spectrometer (Methods, Fig. 1b ). The DF scattered-light spectrum of the uncoated (that is, ‘bare’) AgNPA/Ag metasurface displayed a single peak occurring at 400 nm with a shoulder at ∼ 430 nm ( Fig. 1f ), which, since this peak was not present in the scattered-light spectrum of the bare planar Ag film, arose from a plasmonic resonance of the AgNPA. When a P3HT absorber coating was applied to the AgNPA/Ag metasurface, a new peak emerged at 670 nm with a shoulder ∼ 585 nm ( Fig. 1f,g ). This scattering peak was an unexpected result and occurred just red-shifted from the absorption edge of the P3HT coating ( Supplementary Fig. 5a ). Interestingly, the P3HT-coated planar Ag film also displayed this scattering peak ( Fig. 1f,h ), although the peak wavelength occurred at 655 nm and the intensity was lower compared with the coated metasurface. Scattered-light spectra of absorber-coated planar Ag films To investigate whether this new scattering peak occurred ubiquitously for absorber coatings, we conducted DF scattered-light spectroscopy on planar Ag films with various organic semiconductor coatings ( Fig. 2a ). The scattering spectra showed peaks occurring at wavelengths red shifted from the absorption edge for only certain coatings, particularly those coatings with large lateral feature sizes ( ∼ 100 to 350 nm) or high surface roughness (greater than ∼ 1 nm r.m.s; Fig. 2 ). We attributed the scattering peak observed for coatings with more irregular surfaces to Mie scattering by nanoscale surface features in the organic material modified by its absorption (that is, Mie-‘absorption-induced scattering,’ or Mie-AIS), which we have reproduced through simulations ( Supplementary Fig. 6 ). Additional coated planar Ag films which did not exhibit this Mie-AIS peak (because the coatings had very planar surfaces) are shown in Supplementary Fig. 7 . 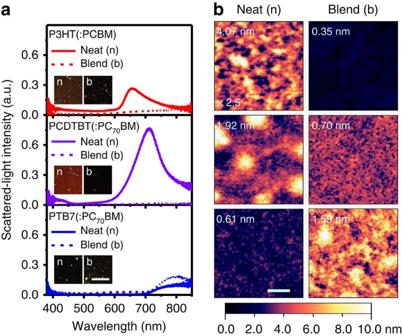Figure 2: Mie-absorption-induced scattering in absorber-coated planar Ag films. (a) DF scattered-light spectra of various neat conjugated polymer (n, solid lines) and polymer:fullerene blend (b, dashed lines) coatings on planar Ag substrates. Insets are true-colour DF images of the coatings on planar Ag substrates and were captured from regions where the DF spectra were acquired. All images are on the same length scale (scale bar, 100 μm, and is shown for PTB7:PC70BM/Ag). (b) AFM surface topography of planar Ag substrates with neat polymer and polymer:fullerene blend coatings corresponding to those in (a). Root-mean-square (r.m.s.) surface roughness values are shown on each image; all images are on the same length scale (scale bar, 500 nm, and is shown for neat PTB7) and height intensity scale, except for neat P3HT (height intensity values are 2.5 × the values on the height scale bar). Figure 2: Mie-absorption-induced scattering in absorber-coated planar Ag films. ( a ) DF scattered-light spectra of various neat conjugated polymer (n, solid lines) and polymer:fullerene blend (b, dashed lines) coatings on planar Ag substrates. Insets are true-colour DF images of the coatings on planar Ag substrates and were captured from regions where the DF spectra were acquired. All images are on the same length scale (scale bar, 100 μm, and is shown for PTB7:PC 70 BM/Ag). ( b ) AFM surface topography of planar Ag substrates with neat polymer and polymer:fullerene blend coatings corresponding to those in (a). Root-mean-square (r.m.s.) surface roughness values are shown on each image; all images are on the same length scale (scale bar, 500 nm, and is shown for neat PTB7) and height intensity scale, except for neat P3HT (height intensity values are 2.5 × the values on the height scale bar). Full size image Scattered-light spectra of absorber-coated metasurfaces Next, we investigated how changing the absorber coating affected the scattering from AgNPA/Ag metasurfaces. Fig. 3a shows both empirical and simulated DF scattered-light spectra for AgNPA/Ag metasurfaces with various coatings (Methods). For bare AgNPA/Ag, a scattering peak was observed in the simulated spectrum at 360 nm, and was attributed to coupled transverse LSPRs of the AgNPs through analysis of the electric field profiles (Mode I; Fig. 3c ). A shoulder was observed at ∼ 390 nm, and was attributed to a hybrid SPP mode between the AgNPA and the Ag film (Mode II; Fig. 3d ), as evidenced from simulated polarization- and angle-dependent scattering spectra ( Supplementary Fig. 8a ) [33] . When coated by absorbers, the scattering spectra of all AgNPA/Ag metasurfaces were split with distinct short ( ∼ 300 to 500 nm) and long ( ∼ 650 to 900 nm) wavelength scattering regimes ( Fig. 3a ). By interpreting electric field profiles and the scattered-light spectrum of a transparent-polymer (that is, poly(methyl methacrylate) (PMMA))-coated AgNPA/Ag metasurface ( Fig. 3b ), the short wavelength scattering was attributed to LSPRs with contributions from coupled transverse LSPRs (Mode I) in addition to multipolar (Mode III) and transverse dipolar (Mode IV) LSPR modes ( Fig. 3a,c,e,f , Supplementary Fig. 9 ). PCDTBT and PTB7 had a dip in the short wavelength scattering due to higher-energy excitonic absorption transitions of the polymers [34] , [35] ( Supplementary Fig. 5a ). The scattering from LSPRs was lower in intensity for the polymer:fullerene blends than for the neat conjugated polymers due to absorption from the fullerene derivatives at wavelengths between 300 and 500 nm ( Supplementary Fig. 5b,c ). The neat fullerene derivatives had similar scattering behaviour to a dielectric coating with refractive index, n , of 2.0 ( Fig. 3b ), due to the higher refractive indices of PCBM and PC 70 BM throughout most of the visible spectrum ( Supplementary Fig. 5c ). However, since PC 70 BM absorbed strongly in the 400–600 nm wavelength range, LSPR scattering was partially absorbed by PC 70 BM. There was relatively good agreement between the simulated and empirical scattering data for the LSPR modes. 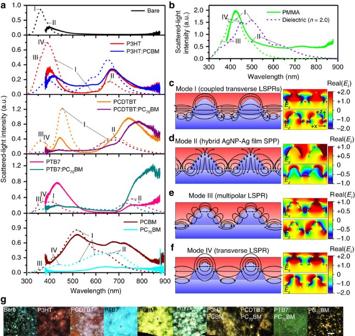Figure 3: Backscattered-light spectra for various absorber coatings. (a,b) Experimental and simulated scattered-light spectra for: AgNPA/Ag metasurfaces with and without various absorber coatings (a) and dielectric-coated AgNPA/Ag metasurfaces (b). Solid lines represent empirical DF spectra, and dashed lines represent finite-difference time-domain (FDTD) simulations of the backscattered spectra. Note that the experimental set-up was limited to a wavelength range of approximately 380–860 nm. (c–f) Schematic depictions of electric field lines and charge distributions (+ and−represent regions of positive and negative charge accumulation, respectively) for the various modes supported by a dielectric (n=2.0)-coated AgNPA/Ag metasurface. Note that the schematics were created based on vector plots of the total electric field and the electric field amplitude profiles (shown to the right of the schematics). The Roman numerals in (a,b) refer to the mode types as referenced in (c–f) and were assigned by analysing the electric field vector plots and amplitude profiles for each peak. The modes occurred at the same or very similar wavelengths between neat conjugated polymers and polymer:fullerene blends and so were only labelled for the simulated spectra of neat conjugated polymers. (g) True-colour DF images of the regions from which corresponding spectra were obtained (regions indicated by small rectangles), all images are on the same length scale (scale bar, 50 μm, and is shown for the PC70BM coating). Figure 3: Backscattered-light spectra for various absorber coatings. ( a,b ) Experimental and simulated scattered-light spectra for: AgNPA/Ag metasurfaces with and without various absorber coatings ( a ) and dielectric-coated AgNPA/Ag metasurfaces ( b ). Solid lines represent empirical DF spectra, and dashed lines represent finite-difference time-domain (FDTD) simulations of the backscattered spectra. Note that the experimental set-up was limited to a wavelength range of approximately 380–860 nm. ( c – f ) Schematic depictions of electric field lines and charge distributions (+ and − represent regions of positive and negative charge accumulation, respectively) for the various modes supported by a dielectric ( n =2.0)-coated AgNPA/Ag metasurface. Note that the schematics were created based on vector plots of the total electric field and the electric field amplitude profiles (shown to the right of the schematics). The Roman numerals in ( a , b ) refer to the mode types as referenced in ( c – f ) and were assigned by analysing the electric field vector plots and amplitude profiles for each peak. The modes occurred at the same or very similar wavelengths between neat conjugated polymers and polymer:fullerene blends and so were only labelled for the simulated spectra of neat conjugated polymers. ( g ) True-colour DF images of the regions from which corresponding spectra were obtained (regions indicated by small rectangles), all images are on the same length scale (scale bar, 50 μm, and is shown for the PC 70 BM coating). Full size image In the long-wavelength regime, the empirically obtained scattering exhibited different behaviour depending on the coating. With P3HT, PTB7 and P3HT:PCBM coatings, a peak occurred at the absorption edge of the coating (670 nm for P3HT and P3HT:PCBM, 756 nm for PTB7). This peak occurred at very similar wavelengths to the Mie-AIS peak observed for absorber-coated planar Ag films; however, unlike Mie-AIS, nanoscale surface roughness on the absorber coating was not the primary cause of this scattering peak since the peak was observed in simulated data for coated metasurfaces, even with a planar organic-air interface (Methods). The electric field profiles, in addition to the simulated scattered-light spectrum of a high-refractive-index ( n =2.0) dielectric-coated AgNPA/Ag metasurface ( Fig. 3b ), revealed that this long-wavelength scattering arose predominantly from the hybrid AgNP-Ag film SPP (Mode II; Fig. 3d ). The scattering peak was pinned just beyond the absorption edge wavelength of the organic semiconductor due to the large increase in refractive index and significant drop in absorption of the coating ( Supplementary Fig. 5a,b ). Since this scattering arose from the collective response of plasmonic modes modified by absorption transitions of the coatings, it is called ‘plasmon-AIS.’ Plasmon–AIS peaks were observed for all absorber-coated metasurfaces and followed the absorption edge of the coatings. We will discuss the physical origin of AIS extensively in the proceeding section. For P3HT- and P3HT:PCBM-coated metasurfaces, there was an additional plasmon–AIS shoulder at ∼ 580 nm, which arose predominantly from the combined response of the Mode I LSPR and the increased refractive index due to the S 0 →S 1 0–1 singlet exciton vibronic absorption in P3HT ( Supplementary Fig. 5a ). For the PCDTBT-, PCDTBT:PC 70 BM- and PTB7:PC 70 BM-coated metasurfaces, there were two distinct components observed empirically for the long-wavelength scattering regime: one component occurred just beyond the absorption edge wavelength of the coatings (665 nm for PCDTBT and PCDTBT:PC 70 BM; 772 nm for PTB7:PC 70 BM) due to plasmon–AIS, and another broader and more intense component occurred at even longer wavelengths (740 nm for PCDTBT; 780 nm for PCDTBT:PC 70 BM; ≥845 nm for PTB7:PC 70 BM). Since the broader, more intense component of the long-wavelength peak occurred for absorber-coated AgNPA/Ag metasurfaces, but not for absorber-coated AgNPA/glass ( Supplementary Fig. 10 ), and this component appeared to be broadband, based on scattering from PMMA-coated AgNPA/Ag metasurfaces ( Fig. 3b ; note the elevated baseline relative to the simulated spectrum), we hypothesized that out-coupled SPPs contributed to this scattering. This long-wavelength scattering component was not present in the backscattered simulations and it occurred empirically only for certain coatings. Furthermore, there were no apparent correlations between the occurrence of the long-wavelength scattering and the surface morphology of the coated AgNPA/Ag metasurfaces ( Supplementary Fig. 4 ). The origins of the long-wavelength contribution will be discussed in greater detail in the following sections. Physical origin of AIS AIS was observed for scattering modes, whether plasmonic (that is, plasmon–AIS, Fig. 3a ) or non-plasmonic (for example, Mie-AIS, Fig. 2a ; see also Supplementary Fig. 11 ), in the presence of an absorber and followed the absorption edge wavelength of the coating. In addition, for AIS, the scattering object required close proximity with the absorber, as AIS was not present when a non-absorptive spacer layer was inserted between the scattering object and absorber coating ( Supplementary Fig. 12 ). We also observed that, although absorber-coated non-plasmonic scatterers gave rise to AIS peaks (for example, Ni or PMMA NPAs— Supplementary Fig. 11a ), plasmonic scatterers resulted in more intense AIS, with AIS peak intensity increasing with better spectral overlap between the LSPR of the metal NPA and the absorption edge of the coating ( Supplementary Fig. 11 , Supplementary Table 1 ). To further elucidate the physical origin of AIS, we varied the NPA period for absorber-coated AgNPA/Ag metasurfaces in electromagnetic simulations ( Fig. 4 ). For periods of ∼ 150 nm, P3HT-coated AgNPA/Ag metasurfaces displayed two dominant scattering peaks: a broad peak ( ∼ 390 nm) composed of Mode I, III and IV LSPRs, and the plasmon–AIS peak ( ∼ 660 nm; Fig. 4a ). For periods ≥250 nm, two branches of the long-wavelength peak were observed: one dispersive, which was attributed to the Mode II hybrid NP-film SPP (based on its presence for the uncoated and dielectric-coated AgNPA/Ag metasurfaces; Fig. 4b,c , Supplementary Fig. 14 ), and one non-dispersive, corresponding to plasmon–AIS arising from the Mode I LSPR. Thus, plasmon–AIS peaks had contributions from both localized and propagating surface plasmon modes (that is, Modes I and II, respectively), which was also supported by excitation polarization-dependent simulations ( Supplementary Fig. 15 ). Furthermore, isolated metal nanoparticles in the presence of a P3HT coating still displayed an AIS peak ( Supplementary Fig. 16 ) arising from a transverse LSPR (Mode IV). Note that for a P3HT-coated glass NPA on a glass substrate, Mie-AIS was observed, which was non-dispersive with array period ( Fig. 4d ). 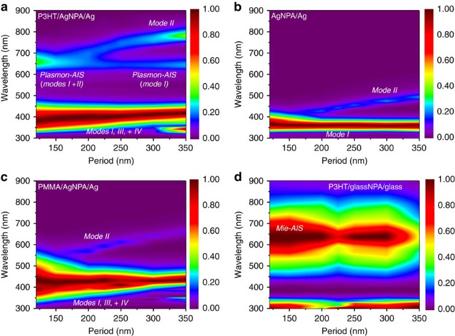Figure 4: The effect of array period on scattered-light spectra. (a) Normalized, simulated scattered-light spectra for P3HT/AgNPA/Ag metasurface as a function of array period, where the different scattering mode types are shown in addition to the plasmon–AIS mode. (b,c) Normalized, simulated scattered-light spectra as a function of array period for bare (b) and PMMA-coated (c) AgNPA/Ag metasurfaces, showing the localized and dispersive modes. (d) Normalized, simulated scattered-light spectra for P3HT/glass NPA/glass as a function of array period, where the Mie-AIS peak is labelled. Note that for (d), the absolute intensities of the scattering peaks are ≥1,000 a.u. smaller than the scattering from (a–c) (seeSupplementary Fig. 13for absolute scattering intensity plots). Note that a course mesh (2.0 nm) was used for these simulations; all other simulation parameters were the same as described in Methods. Figure 4: The effect of array period on scattered-light spectra. ( a ) Normalized, simulated scattered-light spectra for P3HT/AgNPA/Ag metasurface as a function of array period, where the different scattering mode types are shown in addition to the plasmon–AIS mode. ( b , c ) Normalized, simulated scattered-light spectra as a function of array period for bare ( b ) and PMMA-coated ( c ) AgNPA/Ag metasurfaces, showing the localized and dispersive modes. ( d ) Normalized, simulated scattered-light spectra for P3HT/glass NPA/glass as a function of array period, where the Mie-AIS peak is labelled. Note that for ( d ), the absolute intensities of the scattering peaks are ≥1,000 a.u. smaller than the scattering from ( a – c ) (see Supplementary Fig. 13 for absolute scattering intensity plots). Note that a course mesh (2.0 nm) was used for these simulations; all other simulation parameters were the same as described in Methods. Full size image Therefore, the aforementioned results demonstrate that the physical origin of AIS is electromagnetic coupling between the optical transitions of an absorber material and scattering modes, regardless of whether the scattering modes are plasmonic, localized or collective in origin. The general requirements for AIS to be observed are: (1) the presence of a scattering object and an absorber material; (2) spectral overlap between the scattering mode(s) and absorber optical transitions; and (3) close proximity between the scattering object and absorber material. Extent of SPP out-coupling To determine the origin of the longer-wavelength (that is, 740–900 nm) scattering component, we conducted additional FDTD electromagnetic simulations in which we studied the transmission through two 2D monitors oriented normal to the substrate plane (that is, ‘vertical monitors’) placed at a distance 100 nm in front of and behind a cluster of AgNPs (Methods and Fig. 5b , inset). For P3HT:PCBM-coated AgNPA/Ag, transmission through the vertical monitors did not match the empirical long-wavelength scattering well for wavelengths greater than ∼ 675 nm ( Fig. 5b ). The plasmon–AIS peak was observed through the vertical simulation monitors at 650 nm along with an additional mode with a peak at 770 nm. The transmission through the vertical monitors did, however, match the empirical scattered-light spectrum well for the PTB7:PC 70 BM coating ( Fig. 5c ). The spectrally resolved electric field profiles ( Fig. 5a ) revealed that the plasmon–AIS peak was dominated by in-plane electric field components ( E x ), whereas the long-wavelength component (at 770 nm) was dominated by out-of-plane electric field components ( E z ) with the fields bound tightly to the P3HT:PCBM–Ag interface (see Supplementary Figs 17 and 18 for additional field profiles), suggesting that the long-wavelength scattering component observed empirically for certain coatings (for example, PTB7:PC 70 BM) arose from an out-coupled SPP mode. In addition, angle-dependent empirical scattering spectra support this assignment ( Supplementary Figs 19 and 20 ). However, since SPPs were not out-coupled by the AgNPs in the simulations (that is, no long-wavelength scattering peak observed with the back-scattered monitor), we attribute the SPP out-coupling that occurred for certain coatings empirically to physical properties of the coating itself that were not accounted for in simulations. The AgNPs, while not causing out-coupling of SPPs, caused near-field excitation (that is, in-coupling) to the SPPs (Mode V; Fig. 5e and Supplementary Fig. 18 ). 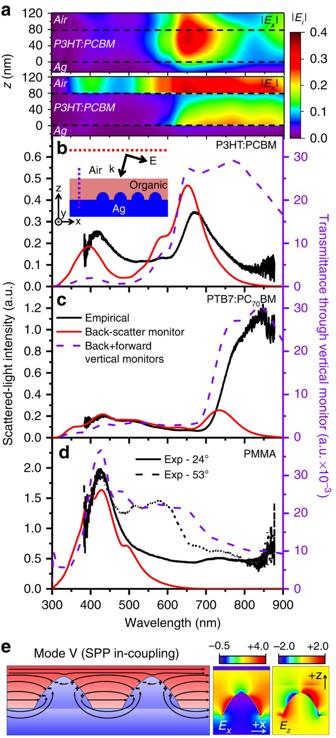Figure 5: Out-coupling of surface plasmon polaritons. (a) Spectral in-plane (Ex) and out-of-plane (Ez) electric field distributions through the forward vertical monitor located 100 nm away from the nearest AgNP for P3HT:PCBM-coated AgNPA/Ag metasurface. (b–d) Empirical and simulated scattered-light spectra (solid lines) and simulated transmission through the vertical monitors (dashed lines) for P3HT:PCBM (b), PTB7:PC70BM (c), and PMMA (d) coatings. Note that the empirical spectra in (b,c) were obtained at an excitation/collection angle of 24°. Inset in (b) shows a schematic of a coated AgNPA/Ag metasurface in which the locations of the backscattered power monitor (red dotted line) and vertical power monitor (purple dotted line) are indicated. (e) Schematic depiction of electric field lines and charge distributions within the near-field of AgNPs that in-couple light to an SPP. Shown to the right of the schematic are real components of the electric field amplitude for the mode. Figure 5: Out-coupling of surface plasmon polaritons. ( a ) Spectral in-plane ( E x ) and out-of-plane ( E z ) electric field distributions through the forward vertical monitor located 100 nm away from the nearest AgNP for P3HT:PCBM-coated AgNPA/Ag metasurface. ( b – d ) Empirical and simulated scattered-light spectra (solid lines) and simulated transmission through the vertical monitors (dashed lines) for P3HT:PCBM ( b ), PTB7:PC 70 BM ( c ), and PMMA ( d ) coatings. Note that the empirical spectra in ( b , c ) were obtained at an excitation/collection angle of 24°. Inset in ( b ) shows a schematic of a coated AgNPA/Ag metasurface in which the locations of the backscattered power monitor (red dotted line) and vertical power monitor (purple dotted line) are indicated. ( e ) Schematic depiction of electric field lines and charge distributions within the near-field of AgNPs that in-couple light to an SPP. Shown to the right of the schematic are real components of the electric field amplitude for the mode. Full size image For PMMA/AgNPA/Ag, broadband SPP modes were also observed through the vertical monitors in addition to LSPR modes at ∼ 430 nm ( Fig. 5d ). Excitation at a large incident angle (53°) in the experiment for the PMMA/AgNPA/Ag revealed some of the simulated peaks observed from the vertical monitors, supporting the hypothesis that the broadband scattering arose from out-coupled SPPs. Therefore, it was expected that broadband SPPs were also supported by absorber-coated AgNPA/Ag, but, for wavelengths within the absorption bands of the coatings, SPPs were absorbed. Hence, we hypothesize that there should be broadband absorption enhancement in the coated metasurface due to a combination of LSPR, broadband SPP, and plasmon–AIS modes. Polarization-dependent reflectance measurements (70° incident angle) for absorber-coated Ag and AgNPA/Ag substrates showed that under transverse magnetic-polarized excitation, there was indeed broadband enhancement in the extinction spectra ( Supplementary Fig. 21 ), supporting our hypothesis. Influence of AgNPA/Ag metasurfaces on polymer crystallinity Although all organic semiconductor coated-AgNPA/Ag metasurfaces supported SPPs, as shown above, only certain coatings out-coupled SPPs well to the far-field in experiments, whereas the other coatings trapped SPPs more efficiently. Since we did not observe a correlation between absorber-coating surface morphology and SPP out-coupling ( Supplementary Fig. 4 ), we chose to investigate the crystallinity and molecular orientation of the organic absorber coatings using grazing-incidence wide-angle X-ray scattering (GIWAXS; Supplementary Figs 22–25 ). Fig. 6a–c shows the expected crystal lattice spacings in the [100] and [010] directions (assigned to the distance between two adjacent backbone chains, and to the π – π stacking distance, respectively) for each neat conjugated polymer [36] , [37] , [38] , [39] . Line profiles were taken either in the out-of-plane ( q z ) or the in-plane ( q r ) direction depending on which direction the dominant scattering peak was oriented for each polymer ( Supplementary Fig. 22 ). Overall, P3HT, P3HT:PCBM and PTB7 coatings had a higher degree of crystallinity compared with the other coatings, based on (100) reflection intensities, regardless of the substrate type. Fig. 6d–f shows 1D GIWAXS line profiles for the three neat polymers on glass, planar Ag and AgNPA/Ag substrates. The intensities of the (100) peak for each of the neat polymers were reduced for AgNPA/Ag substrates relative to planar Ag or glass substrates. This trend held for the other polymer reflections for both in-plane and out-of-plane directions ( Supplementary Fig. 24a–c ), suggesting that there was a reduction in the crystallinity of neat polymers when coated onto AgNPA/Ag substrates. This trend did not hold for polymer:fullerene blends ( Fig. 6g–i ). For P3HT:PCBM ( Fig. 6g ), the out-of-plane (100) P3HT peak was more intense for the AgNPA/Ag substrate relative to both Ag and glass substrates. However, the in-plane (100) peak was reduced for the AgNPA/Ag substrate ( Supplementary Fig. 24d ), indicating that for P3HT:PCBM, the AgNPA oriented the P3HT molecules in a more edge-on configuration relative to planar Ag or glass substrates. Since the PCDTBT:PC 70 BM blend was amorphous, there was not a notable trend for the PCDTBT reflections for the three substrates ( Fig. 6h ). For PTB7:PC 70 BM, the in-plane (100) peak was more intense for the AgNPA/Ag substrate relative to the blend on both planar Ag and glass ( Fig. 6i ), as was the in-plane (010) reflection ( Supplementary Fig. 24f ), indicating that the AgNPA increased the overall crystallinity of the PTB7 in the blend. 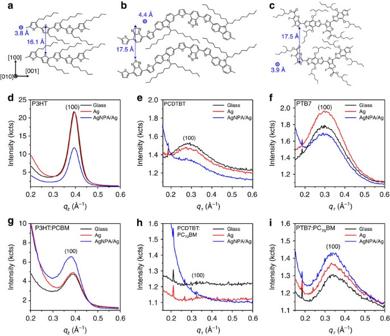Figure 6: Grazing-incidence wide-angle X-ray scattering measurements. (a–c) Molecular structures and expected physical distances of P3HT (5 monomer repeat units shown per chain segment in (a)), PCDTBT (two monomer repeat units shown per chain segment in (b)), and PTB7 (two monomer repeat units shown per chain segment in (c)). Two adjacent chain segments are shown for each polymer. Note that the [100] direction corresponds to the distance between adjacent backbone chains (that is, intermolecular side-chain packing direction) and the [010] direction corresponds to theπ–πstacking direction. (d–i) GIWAXS from polymer (d–f) and polymer:fullerene (g–i) thin-film coatings on various substrates. (d,g) Out-of-plane (qz) line scans extracted atqr=0 for P3HT (d) and P3HT:PCBM (g) coatings, where the (100) reflections are shown. (e,f,h,i) In-plane (qr) line profiles extracted atqz=0 for PCDTBT (e), PTB7 (f), PCDTBT:PC70BM (h), and PTB7:PC70BM (i) coatings, where the (100) reflections are shown. Figure 6: Grazing-incidence wide-angle X-ray scattering measurements. ( a – c ) Molecular structures and expected physical distances of P3HT (5 monomer repeat units shown per chain segment in ( a )), PCDTBT (two monomer repeat units shown per chain segment in ( b )), and PTB7 (two monomer repeat units shown per chain segment in ( c )). Two adjacent chain segments are shown for each polymer. Note that the [100] direction corresponds to the distance between adjacent backbone chains (that is, intermolecular side-chain packing direction) and the [010] direction corresponds to the π – π stacking direction. ( d – i ) GIWAXS from polymer ( d – f ) and polymer:fullerene ( g – i ) thin-film coatings on various substrates. ( d , g ) Out-of-plane ( q z ) line scans extracted at q r =0 for P3HT ( d ) and P3HT:PCBM ( g ) coatings, where the (100) reflections are shown. ( e , f , h , i ) In-plane ( q r ) line profiles extracted at q z =0 for PCDTBT ( e ), PTB7 ( f ), PCDTBT:PC 70 BM ( h ), and PTB7:PC 70 BM ( i ) coatings, where the (100) reflections are shown. Full size image The differences in the observed trends between polymer:fullerene blends could have arisen from differences in: molecular orientation of the polymer crystallites (edge-on for P3HT, face-on for PTB7); molecular weights of the polymers; polymer:fullerene blend ratios; solvents used for the deposition; or the identity of the fullerene derivatives. Further studies are necessary to determine if AgNPA/Ag metasurfaces impact polymer:fullerene morphology in a predictable manner. In the Discussion section, we correlate the observed differences in crystallinity between the coatings to the extent of SPP out-coupling observed empirically in scattered-light spectra. Note: while outside the scope of this study, improvement of the order and alignment of the polymers in the polymer:fullerene blends could be useful for improving the charge extraction efficiency for BHJ-OPV devices incorporating metasurfaces as electrodes. However, since charge extraction is improved for the face-on orientation [39] , [40] , metasurfaces which re-orient the molecules in the face-on direction would be preferred. Since PTB7 crystallizes in the face-on direction, the AgNPA may be more useful for improving the charge extraction efficiency from PTB7-based BHJ-OPVs compared to P3HT- and PCDTBT-based BHJ-OPVs. Absorption spectra of absorber-coated AgNPA/Ag metasurfaces To determine how effectively the various optical modes (that is, LSPRs, plasmon–AIS, and SPPs) improved absorption in the coated AgNPA/Ag metasurfaces, integrating sphere reflectance measurements were employed (Methods); Fig. 7a . Compared with bare planar Ag (which exhibited minimal absorption) and bare AgNPA/Ag (where part of the LSPR was observed at ∼ 370 nm), absorption increased on coating with a transparent PMMA film, which we attribute to red-shifts and trapping of LSPRs and SPPs due to the higher refractive index environment. For conjugated polymer:fullerene coatings, absorption was improved between 360 and 450 nm, where LSPRs had the greatest contribution; PCDTBT:PC 70 BM and PTB7:PC 70 BM both displayed broadband absorptance enhancement, especially the latter coating. The greatest enhancement occurred at wavelengths >630 nm for P3HT:PCBM and >700 nm for PCDTBT:PC 70 BM and PTB7:PC 70 BM, attributed to SPPs, with enhancement factors reaching nearly 6 at 800 nm for PTB7:PC 70 BM. Although these enhancement factors were reasonably large, parasitic absorption by the Ag or AgNPA could not be ruled out from the integrating sphere absorption measurements. 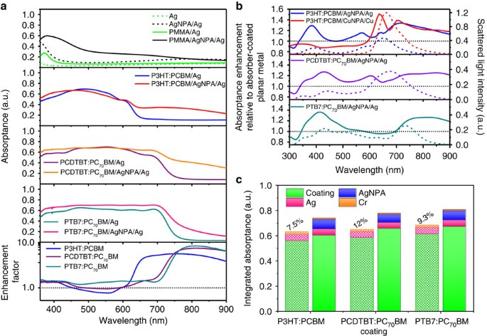Figure 7: Absorption measurements and simulations. (a) Integrating-sphere absorptance spectra for polymer:fullerene films coated on optically-thick Ag and AgNPA/Ag films. Bottom panel of (a) shows the absorptance enhancement factor of the polymer:fullerene-coated AgNPA/Ag metasurface relative to the polymer:fullerene-coated Ag substrate (vertical axis increment spacing is 1). (b) Simulated absorptance enhancement in the coating for polymer:fullerene-coated AgNPA/Ag or CuNPA/Cu metasurfaces relative to polymer:fullerene-coated planar Ag or Cu substrates, respectively (solid lines). The simulated scattered-light spectra are shown as dashed lines for comparison. (c) Integrated absorptance weighted by the AM1.5 solar spectrum for each layer. The solid bars represent the AgNPA/Ag substrates, and the cross-hatched bars represent the planar Ag substrates. The numbers over the planar polymer:fullerene bars indicate the total percent absorptance change in the absorber coating for AgNPA/Ag substrates compared to planar Ag substrates, integrated over all wavelengths. Figure 7: Absorption measurements and simulations. ( a ) Integrating-sphere absorptance spectra for polymer:fullerene films coated on optically-thick Ag and AgNPA/Ag films. Bottom panel of ( a ) shows the absorptance enhancement factor of the polymer:fullerene-coated AgNPA/Ag metasurface relative to the polymer:fullerene-coated Ag substrate (vertical axis increment spacing is 1). ( b ) Simulated absorptance enhancement in the coating for polymer:fullerene-coated AgNPA/Ag or CuNPA/Cu metasurfaces relative to polymer:fullerene-coated planar Ag or Cu substrates, respectively (solid lines). The simulated scattered-light spectra are shown as dashed lines for comparison. ( c ) Integrated absorptance weighted by the AM1.5 solar spectrum for each layer. The solid bars represent the AgNPA/Ag substrates, and the cross-hatched bars represent the planar Ag substrates. The numbers over the planar polymer:fullerene bars indicate the total percent absorptance change in the absorber coating for AgNPA/Ag substrates compared to planar Ag substrates, integrated over all wavelengths. Full size image Electromagnetic simulations were employed to determine how much of the enhanced absorption in the presence of the AgNPA was beneficial (that is, absorbed by the absorber coating alone) as opposed to parasitic (that is, absorbed by the AgNPA, Ag or Cr layers); see Fig. 7b,c . The simulations showed that absorption enhancement in the coatings was indeed broadband, although different spectral regimes were enhanced to a larger degree than others. In general, the maximum absorptance enhancement for all three coatings occurred at wavelengths corresponding to the LSPR peaks from the AgNPA ( ∼ 340 to 480 nm), with a maximum enhancement factor of 1.36 observed in this wavelength range for PTB7:PC 70 BM/AgNPA/Ag relative to PTB7:PC 70 BM/Ag ( Fig. 7b ). The absorptance enhancement remained large for wavelengths beyond the absorption edge of each of coating, with enhancement factors reaching values up to 1.34 for P3HT:PCBM/AgNPA/Ag at 710 nm (attributed to coupling into SPPs) relative to P3HT:PCBM/Ag. Near the plasmon–AIS peak wavelength, particularly for P3HT:PCBM and PCDTBT:PC 70 BM coatings, dips in the coating absorptance enhancements occurred, indicating increases in scattering losses and/or parasitic absorption loss in the metal. However, on either side of the plasmon–AIS peak wavelength, there were peaks in the absorptance enhancement, confirming that there was electromagnetic coupling between the absorber optical transition and scattering mode [15] . The absorptance enhancement dip was not observed for the PTB7:PC 70 BM coating because of the poor spectral overlap between the absorption edge and the scattering modes (note the lower intensity of the plasmon–AIS peak for PTB7:PC 70 BM compared with the other two coatings). When the LSPR of the metasurface was tuned to spectrally overlap with the absorption edge of the coating (that is, by switching from a AgNPA/Ag metasurface to a CuNPA/Cu metasurface with a P3HT:PCBM coating), the absorptance enhancement at the absorption edge of the coating was significantly increased (to a value of ∼ 1.5) relative to P3HT:PCBM/Cu, and the absorptance enhancement had very well-defined peaks on either side of the plasmon–AIS peak wavelength, suggesting stronger coupling between the P3HT:PCBM optical transitions with the LSPR of the CuNPA/Cu metasurface. However, for other spectral regimes, the absorptance in the P3HT:PCBM coating was reduced relative to P3HT:PCBM/Cu. Thus, although the absorption enhancement was maximized by overlapping the LSPR with the absorption edge, the absorption in the coating was reduced relative to planar Cu substrates for other spectral regimes. Overlapping the LSPR with the absorption edge is beneficial when strong absorption in the coating is desired at particular wavelengths, such as for photodetectors or sensors, but for broadband absorption enhancement, spectrally separating the LSRP from the absorption edge is more beneficial. Note that absorptance in the metal NPA/metal film was also enhanced at these wavelengths ( Supplementary Figs 26e and 27b ), which could be of interest for plasmon–enhanced hot carrier generation [41] . Figure 7c shows the computed integrated absorptance weighted by the AM1.5 spectrum in each layer for the AgNPA/Ag substrates and planar Ag substrates. The total parasitic absorptance in the Ag and Cr materials for the planar substrates was less than 7 % for all active layer coatings and up to 14 % for AgNPA/Ag with a P3HT:PCBM coating. However, even though parasitic absorption increased in the presence of AgNPA/Ag, total coating absorption was improved for all coating materials from absorptance values between 56 and 62 % for the coated-planar Ag substrates to absorptance values between 60 and 67 % for the coated-AgNPA/Ag metasurfaces. LSPRs improved absorptance in the coating (by up to 6 %) to a larger degree than in the metal (3 %), whereas plasmon–AIS and SPPs increased absorptance in the metal (by up to 1.6 %) to a larger degree than in the coating ( Supplementary Table 2 ). This was attributed to very small or negligible absorption coefficients of the organic semiconductors in the wavelength regimes of plasmon–AIS and SPPs compared to those in the wavelength regimes of the LSPRs, coupled with the fact that absorptance enhancement had both dips and peaks in the wavelength regime of plasmon–AIS. Several conclusions can be drawn from the results of the scattered-light spectroscopy, electromagnetic simulations, surface morphology and crystallinity studies for the various organic semiconductor absorber coatings and are schematically represented in Fig. 8a–c . For absorber coatings on planar Ag, nanoscale surface features in the coating resulted in Mie-AIS occurring at wavelengths just red-shifted from the absorption edge of the coating. This may be of interest for improved light trapping in photovoltaic applications—in cases where nanoscale surface roughness does not degrade other performance parameters of a device, it may be beneficial to incorporate some degree of roughness in thin-film absorber layers to help scatter sub-bandgap light where absorption is weakest. 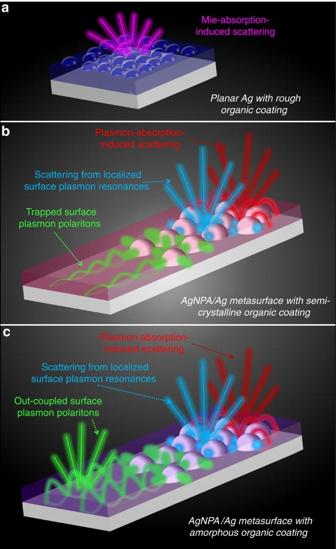Figure 8: Scattering modes supported by absorber-coated plasmonic metasurfaces. (a) The organic semiconductor-coated planar Ag film has been shown to only support Mie-AIS for organic coatings exhibiting high degrees of nanoscale surface features. (b,c) The organic semiconductor-coated AgNPA/Ag metasurfaces have been shown to support various LSPR, plasmon–AIS and SPP modes. While the LSPR and plasmon–AIS modes backscatter for all absorber coatings, the SPP mode was trapped for semicrystalline organic absorber coatings (b) and was only scattered to the far field for the amorphous organic absorber-coated metasurfaces (c). Figure 8: Scattering modes supported by absorber-coated plasmonic metasurfaces. ( a ) The organic semiconductor-coated planar Ag film has been shown to only support Mie-AIS for organic coatings exhibiting high degrees of nanoscale surface features. ( b,c ) The organic semiconductor-coated AgNPA/Ag metasurfaces have been shown to support various LSPR, plasmon–AIS and SPP modes. While the LSPR and plasmon–AIS modes backscatter for all absorber coatings, the SPP mode was trapped for semicrystalline organic absorber coatings ( b ) and was only scattered to the far field for the amorphous organic absorber-coated metasurfaces ( c ). Full size image There were three dominant mode types observed for the absorber-coated AgNPA/Ag metasurfaces: LSPRs of individual AgNPs (Modes I, III, and IV in Fig. 3 ) at short wavelengths ( ∼ 350 to 550 nm); plasmon–AIS just red-shifted from the absorption edge of the coatings (arising from both localized (Mode I) and propagating (Mode II) plasmonic modes), and out-coupled SPPs (from Mode V) at wavelengths longer than plasmon–AIS. The plasmonic scattering modes which spectrally overlapped the optical transitions of the absorber (Modes I and II) became pinned to wavelengths just red-shifted from the absorption edge of the absorber, arising from the increased refractive index and minimal absorption from the coating at these wavelengths. This pinning of the plasmonic modes gave rise to plasmon–AIS, which we speculate has been observed indirectly in prior studies of plasmon–enhanced inorganic photovoltaics [42] , [43] , [44] , [45] , plasmonic nanoparticles embedded in organic photovoltaic active layers [46] , [47] , [48] , and organic photovoltaics employing nanostructured back electrodes (similar to the metasurfaces described here) [20] , [49] , [50] , [51] , [52] . In all of these studies, a strong absorption and/or photocurrent enhancement was observed just red-shifted from the absorption edge of the photovoltaic absorber and was primarily attributed to either efficient scattering from dipolar or multipolar LSPRs [42] , [43] , [44] , [45] , [49] , which, in some cases, were shifted by the refractive index of the active layer [20] , [46] , [47] , or excitation of SPPs at these wavelengths [51] , [52] . Since, in this work, we have shown that the physical origin of AIS is electromagnetic coupling between optical transitions of absorber materials and scattering modes, we expect that AIS was present in these and other prior studies and contributed to some extent to the enhanced absorption or photocurrent near the absorption edge of the semiconductors. By comparing empirical scattered-light spectra with GIWAXS results, scattering from out-coupled SPPs was found to be lower in intensity for polymer or polymer:fullerene coatings with higher degrees of crystallinity (P3HT, P3HT:PCBM, PTB7) than for the more amorphous coatings (PCDTBT, PCDTBT:PC 70 BM, PTB7:PC 70 BM). We suggest that semicrystalline coatings trapped SPPs to a greater extent than amorphous coatings due to a combination of: (1) total internal reflection at the absorber–air interface, since semicrystalline materials tend to have higher refractive indices than amorphous materials; (2) more tightly bound, shorter propagation length SPPs, again due to the higher refractive indices of semicrystalline coatings; (3) absorption of long-wavelength SPPs by photoinduced absorption from delocalized polarons in crystalline domains, which is known to occur at ∼ 730 nm for regioregular P3HT [53] , [54] (photoinduced absorption from localized polarons in disordered P3HT domains occurs at ∼ 950 nm (ref. 53 )). Furthermore, SPPs were out-coupled to a greater degree empirically because the simulations did not account for effects such as surface roughness, crystallinity and the conformal nature of the organic coatings, or irregular regions of the metasurface where there were no AgNPs due to imperfections in the fabrication process. In these studies, although amorphous coatings facilitated out-coupling of SPP modes and, hence, their detection by DF spectroscopy, since semicrystalline coatings trapped SPPs better, SPP modes should be more efficiently absorbed by semicrystalline polymers and polymer:fullerene blends. We suggest that if these AgNPA/Ag metasurfaces are employed as electrodes in PLEDs, then amorphous polymer coatings could increase the out-coupling efficiency of emitted light coupled to tightly bound SPP modes, which is a major loss channel in PLED devices [55] . From our results, it is apparent that assessment of the impact of metasurfaces on organic semiconductor morphology and crystallinity should be conducted along with optical studies to fully account for the empirically observed optical properties. Although total integrated absorption enhancements in the organic semiconductor layers were modest using metasurfaces (values as large as 12 %), it is expected that when incorporated into a completed optoelectronic device (that is, addition of charge transport layers, transparent electrode and anti-reflection layers), total absorption could be improved by minimizing reflection losses at the air–polymer:fullerene interface. In addition, although absorption enhancements were large for wavelengths greater than the absorption edge of the polymer:fullerene blends ( Fig. 7b ), the total computed absorptance was still very low for these wavelengths ( ∼ 1% or less). However, empirical studies have demonstrated that there can be significant external quantum efficiency enhancements for sub-bandgap wavelengths (for example, contributing to photoinduced absorption by charge transfer states or polarons [53] , [54] ), suggesting that the optical modes observed through our scattering experiments and simulations could be more beneficial to optoelectronic device performance than predicted by optical absorption simulations alone. This drives the need for electrical and device measurements to fully explore the usefulness of these sub-bandgap optical modes. In summary, large-area metasurfaces composed of Ag nanoparticle arrays on Ag thin films coated with various organic conjugated polymer and polymer:fullerene absorber layers were characterized. Dark-field scattering studies in conjunction with atomic force microscope topography measurements and electromagnetic simulations revealed several optical modes supported by the organic semiconductor-coated metasurfaces: LSPRs; hybrid SPPs between nanoparticles and the underlying metal film; AIS, both from nanoscale organic semiconductor surface features and from coupling of surface plasmon modes to absorbers; and broadband propagating SPP modes. We elucidated the physical origin of the previously unidentified optical mode, AIS, as electromagnetic coupling of absorber optical transitions and scattering modes, regardless of whether the scattering modes are plasmonic, localized or collective in origin. Grazing-incidence X-ray scattering results demonstrated that the crystallinity of neat polymers was reduced in the presence of the metasurface, whereas the alignment of P3HT molecules and the crystallinity of PTB7 molecules in the polymer:fullerene blends were improved in the presence of the metasurface. By correlating polymer crystallinity with scattered-light spectra of the absorber-coated metasurfaces, semicrystalline polymer coatings were found to trap SPP modes better than amorphous polymer coatings. Total absorptance spectra of these structures were determined using using integrating sphere reflectance spectroscopy, and parasitic absorption was separated from absorber coating absorption using electromagnetic simulations. It was found that LSPRs led to the maximal absorption enhancement in the organic coating, although broadband SPPs and plasmon–AIS resulted in improved absorption in the organic coatings, albeit to a lesser degree. We expect that the usefulness of the near- and sub-bandgap optical modes (that is, plasmon–AIS and SPPs) was underestimated by performing optical simulations alone, and could be exploited to a greater extent in completed photovoltaic devices. We foresee that further tuning of the coupling between absorber optical transitions and scattering modes could result in greater absorption enhancements in absorber-coated metasurfaces. Template-based fabrication of plasmonic metasurfaces Glass microscope slides (Fisherbrand, 1 mm thick) were cut into approximately 16 mm × 16 mm segments, which were then sonicated in detergent for 15 min., soaked in a solution of ethanol and concentrated hydrochloric acid (1:1) for 15 min., then soaked in isopropanol for 10 min. before being dried individually using compressed air. The base metal film underlying each of the metallic nanoparticles consisted of 50 nm of Ag on 5 nm of Cr (used as an adhesion layer). To prepare the metal films, cleaned substrates were mounted in the thermal evaporation chamber (Edwards E306A) with a shadow mask used to define metal stripes 1 mm in width and 10 mm in length. The pressure of the chamber was <8 × 10 −6 mbar for both Cr and Ag depositions, and the deposition rate was less than 0.1 nm/s. After each evaporation, the chamber was left to cool for at least 30 min. before venting. To prepare through-hole anodic aluminium oxide (AAO) masks, first AAO nanotemplates (Synkera Inc.) with an average pore diameter of 55 nm and aluminium oxide thickness of ∼ 500 nm (coated on both sides of aluminium) were cut into 15 mm × 10 mm pieces. The back of the nanotemplate was fully protected with epoxy as well as a ∼ 2-mm rim on the front. The exposed AAO layer was etched using NaOH (3 M) for 20 min., then the nanotemplates were subsequently floated on a bath of aqueous FeCl 3 (250 g l −1 ) for ∼ 2 h. to etch the aluminium layer. After, the nanotemplates were immersed into an aqueous H 3 PO 4 (5 % w/w) bath, which was held at 30 °C while stirred at 1,200 r.p.m. The H 3 PO 4 was used to remove the barrier layer and widen the pores of the AAO nanotemplate. The AAO nanotemplates were left in the H 3 PO 4 for between 45 and 55 min., until the pores widened to ∼ 100 nm in diameter as confirmed using scanning electron microscopy (SEM). After, the epoxy layer was removed by immersing the nanotemplates in 5 sequential acetone baths, followed by ethanol and, finally, isopropanol baths. Once prepared, the through-hole AAO nanotemplates were transferred to the metal films. The nanotemplate-covered metal films were mounted in the evaporation chamber and the same shadow masks were used again while evaporating through the nanotemplates, except one of the stripes of the shadow mask was blocked off using Kapton tape for the planar Ag electrode. 60 nm of Ag was deposited through the nanotemplate using the same conditions as for the base metal film deposition. After the deposition, the samples were immersed in a stream of isopropanol to remove the AAO nanotemplate. The samples were then dried using compressed air, and stored in a vacuum desiccator until further characterization or subsequent sample preparation steps. To characterize NP size and coverage, the planar Ag and AgNPA/Ag plasmonic metasurface were imaged using DF microscopy and SEM, with an accelerating voltage of 5.0 kV and a working distance <5 mm. See Supplementary Figs 1 and 2a for additional SEM and DF images of the electrodes. Polymer solution and thin-film preparation Neat polymer solutions were prepared with 10 g l −1 concentration. P3HT (Alfa Aesar, product number: 44745; M w : 30,000–50,000 g mol −1 ; >95 % regioregularity; polydispersity index (PDI)=4.5) and PTB7 (Aldrich, product number: 772410; M w : 80,000–200,000 g mol −1 ; PDI≤3.0) were both separately dissolved in chlorobenzene; PCDTBT (Aldirch, product number: 753998; M w : 20,000–100,000 g mol −1 ; PDI=4.1) was dissolved in o -dichlorobenzene. For the blends, P3HT and PC 60 BM (Aldrich, product number: 684449) in a 1:1 ratio were dissolved in chlorobenzene (20 g l −1 total blend concentration); PCDTBT and PC 70 BM (1-Material, product number OS0633) in a 1:4 ratio were dissolved in o -dichlorobenzene (50 g l −1 total blend concentration); and PTB7 and PC 70 BM in a 1:1.5 ratio were dissolved in a mixture of chlorobenzene and 1,8-diiodooctane (97:3 % v / v ) (25 g l −1 total blend concentration). The P3HT, P3HT:PC 60 BM, PTB7, and PTB7:PC 70 BM solutions were heated to 50 °C and stirred at 1,200 r.p.m. for ∼ 10 min; then were stirred for ∼ 16 h at 1,200 r.p.m. and room temperature. The PCDTBT and PCDTBT:PC 70 BM solutions were heated to 90 °C and stirred at ∼ 1,200 r.p.m. for ∼ 8 h. All solutions were spin-coated at varying speeds to achieve ∼ 80-nm thick films, as confirmed using atomic force microscopy (AFM). See Supplementary Fig. 3 for details on spin-coating conditions and polymer film thickness measurements. Atomic force microscopy A Veeco Digital Instruments Multimode AFM was used for film thickness and surface morphology characterization. The AFM was used in tapping mode, and silicon probes (Bruker, MPP-11100-10) with a nominal tip radius of 8 nm were used for all measurements. All surface morphology scans were acquired over a 2.0 μm × 2.0 μm area with a scan rate of 0.250 Hz and 512 samples/line. The images were flattened using Gwyddion 2.35 software, and root-mean-square (r.m.s) roughness values were determined in the software. Dark-field scattered-light imaging spectroscopy A Nikon Optiphot 66 optical microscope operating in reflection mode was used to locate AgNPA regions. DF images were taken of these regions using a 20 × DF microscope objective and a colour CCD camera. Unless otherwise specified, a halogen lamp (50 W) was used as the illumination source for all DF images and spectra. DF spectra were collected using an Andor Shamrock SR 303i imaging spectrometer. Scattered light from each AgNPA region was excited and collected with a 20 × DF microscope objective (NA=0.40) and the image was directed into the imaging spectrometer. A particular nanoparticle region was selected by imaging through the entrance slit of the spectrometer (an entrance slit width of 250 μm was used, which corresponded to ∼ 10 μm of the sample), and the height of each region was binned to 40 pixels, which corresponded to ∼ 20 μm such that the total area from which spectra were collected was 10 μm × 20 μm (see boxes in Fig. 3g ). DF reflected-light spectra of the selected region (DF sample ) were acquired by inserting an opaque stop in the excitation lamp light path to achieve a hollow cone of illumination ( Fig. 1b ), opening the field and aperture diaphragms fully, and by using an exposure time of 20 s for 6 accumulations using halogen lamp illumination. Background spectra were collected by blocking the light path to the spectrometer and using the same exposure time and accumulations as for the sample . Spectra were normalized to the lamp spectral intensity using DF spectra of a diffuse reflector (Spectraflect, that is, barium sulfate) at the same magnification using an exposure time of 1 s for 6 accumulations (DF diffuse ). A separate background spectrum was taken using the same conditions used for the diffuse reflector . Scattered-light intensity values reported here were calculated using the following equation: The spectrometer was calibrated based on three separate emission lines in a spectrum collected from a Hg vapour lamp. Due to low signal-to-noise ratios, we did not obtain DF scattered-light spectra below 400 nm and above ∼ 800 nm. Integrating sphere absorption measurements The integrating sphere absorption measurements were acquired on an SI Photonics ultraviolet–visible spectrometer (model 440) using halogen lamp illumination (10 W). Samples were prepared as described above, except the underlying Ag film was 150-nm thick to ensure it was optically opaque. AAO nanotemplates were prepared with an area of more than 10 × 10 mm and placed directly on a large-area Ag film to give AgNPA/Ag regions more than 10 × 10 mm in area. Samples were mounted to a 9-mm metallic aperture attached to the port of the integrating sphere, which was coated internally with Spectraflect (that is, barium sulfate). The SI Photonics software automatically determined the exposure time for each spectrum, and 100 spectra were accumulated for each measurement. The reflected light intensity of each sample ( I s ) was normalized to the reflected light intensity of a diffuse reflector ( I 0 ), and the absorptance ( A ) was computed using the equation: A =1− I s / I 0 . Grazing-incidence wide-angle X-ray scattering measurements GIWAXS measurements were performed at the X9 undulator-based beamline at the National Synchrotron Light Source, Brookhaven National Laboratory. The incident X-ray beam energy of 14.1 keV ( λ =0.0879, nm) was collimated using slits and focused onto the sample position using Kirkpatrick–Biaz mirrors, which provided a 100-μm wide × 50-μm high spot at the sample position whose footprint spread along the sample in the direction of propagation of the beam. The sample stage and a 2D charge-coupled device (CCD) detector were located inside a vacuum chamber (pressure ∼ 40 Pa). A rectangular beam stop was positioned just before the CCD to block the primary and the specular reflective beams. All of the measurements reported here were acquired at an incident angle of 0.12° with respect to the sample plane (that is, grazing incidence) and were collected with an acquisition time of 10 s. Data analysis was completed using the view.gtk software developed at the X9 beamline [56] . Backscattered light simulations Full-field electromagnetic simulations were performed using commercially available FDTD software (Lumerical FDTD Solutions). The structures were defined in the software to match the fabricated plasmonic metasurfaces as closely as possible (80 nm polymer or fullerene coating/AgNPA/50 nm Ag/5 nm Cr/glass). The simulated AgNPA was a hexagonally packed array of paraboloids that were created using the equation: which was rotated about the z -axis, where x , y and z are the Cartesian coordinates corresponding to the spatial grid used in the simulations, h was the height of the paraboloids (60 nm), and d was the base diameter of the paraboloids (100 nm). The center-to-center distance between AgNPs (that is, the period) was 150 nm. To simulate backscattered light, the excitation source used was a total-field scattered-field (TFSF) plane wave incident at 15° from the surface normal. Due to the fixed k -vector in the simulations, and since the simulations were broadband, the incident angle of the plane wave actually varied from 10° to 30° from 300 to 900 nm. The TFSF source allowed the separation of the scattered electromagnetic fields from the total electromagnetic fields for the structures under study. The source was injected at a distance of 55 nm above the top of the AgNPA with transverse magnetic polarization. The TFSF source was extended beyond the x and y boundaries of the FDTD simulation region such that the edges of the source extended through the planar Ag region, which was taken as a reference for the subtraction of the total field. The wavelength range of the source was 300–900 nm with 4-nm increments and a source pulse length of 1.995 fs. The FDTD simulation region x , y cross-sectional area was set to 150 × 260 nm with a depth of 2,000 nm in the z direction. The boundary conditions used were perfectly matched layers (PML) in the planes parallel to the substrate ( x – y planes) and Bloch boundary conditions in the two orthogonal planes ( x – z and y – z planes). The number of PML layers was adjusted to achieve total PML reflection of 10 −10 or less. A frequency-domain power monitor was placed 840 nm above the top of the AgNPA and the transmission through this monitor was used as the simulated backscattered spectra. The simulation was stopped either after 100 fs of simulation time or when the fields decayed to less than 5 × 10 −4 of their initial value. A mesh override region was added to cover the TFSF source completely to ensure a constant mesh step size of 0.8 nm throughout the region including the AgNPs in all three spatial directions. The mesh refinement option chosen was ‘conformal variant 1’, and the mesh accuracy was set to 4 outside of the refinement area (only in free space above the structures and in the glass substrate). See Supplementary Fig. 28 for a graphical depiction of the simulation set-up. The optical constants used for the simulations were taken from literature values and are shown in Supplementary Fig. 5 . Surface plasmon polariton simulations For the simulated spectra of the forward- and backward-traveling SPPs, the same general set-up was employed as described for the backscattered light simulations, with the following changes. Supplementary Fig. 29 shows a graphical depiction of the simulation set-up. The FDTD simulation region x , y cross-section was extended to 2,000 × 2,000 nm; the boundary conditions in all directions were set to PML; the TFSF source did not extend beyond the FDTD boundaries, but still was large enough to envelope the seven AgNPs in the one hexagonal unit cell. The mesh override region was also set to 2 nm due to the larger region simulated and the finite computational memory available. Two frequency-domain power monitors were placed at a distance 100 nm in front of and behind the AgNP unit cell in the y – z plane, normal to the thin-film stack. Each of the monitors extended fully through the polymer layer, 25 nm into the Ag film, and 40 nm above the polymer film to collect most of the evanescent fields propagating away from the AgNPs. The transmission through these monitors was summed and reported as the forward+backward vertical monitors in Fig. 5b–d , and the electric field distributions through the forward-traveling vertical monitors were used in Fig. 5a and Supplementary Fig. 17i–n . Another frequency-domain power monitor was placed 115 nm above the top of the polymer coating in the x – y plane, parallel to the sample surface. The electric field distributions in these monitors were reported in Supplementary Fig. 17c–h . Absorption enhancement simulations For the absorption enhancement simulations, the same general set-up was employed as described for the backscattered light simulations, with the following changes. Supplementary Fig. 30 shows a graphical depiction of the simulation set-up. A normal plane wave source was used instead of a TFSF source, which was injected at a distance of 400 nm above the top of the AgNPs and extended beyond the x and y boundaries of the FDTD simulation region. A fully 3D frequency-domain power monitor was placed surrounding the thin-film stack in the z direction and extended beyond the x and y boundaries of the FDTD simulation region. A 3D refractive index monitor was overlaid on the frequency-domain power monitor. The mesh override region remained 0.8 nm, but the fields were sampled every 1.6 nm, and the wavelength increment was increased to 5 nm due to the finite computational memory associated with 3D field and index monitors. Absorption in each layer was calculated using the following equation: where n is the real part of the complex index of refraction, α is the attenuation coefficient (4 πk / λ ), and | E / E 0 | 2 is the normalized electric field intensity squared [57] . The absorption was integrated spatially and normalized to the area illuminated ( S illum ) to obtain the spectral fraction of light absorbed in each layer: The absorption in the active layer was separated from the absorption in the AgNPA by using the refractive index monitor as a reference. Finally, the integrated absorptance in each layer was weighted by the AM1.5 solar spectrum ( P AM1.5 ) and integrated over all wavelengths: FDTD simulations were also conducted for planar Ag electrodes. These simulations were identical to the absorption enhancement simulations containing the AgNPA, except that the AgNPA was removed. Absorption enhancement factors were calculated by dividing absorption in the coating layer on the AgNPA/Ag metasurfaces by the absorption in the coating layer on the planar Ag substrates. How to cite this article: Petoukhoff, C. E. & O’Carroll, D. M. Absorption-induced scattering and surface plasmon out-coupling from absorber-coated plasmonic metasurfaces. Nat. Commun. 6:7899 doi: 10.1038/ncomms8899 (2015).